Extrachromosomal driver mutations in glioblastoma and low-grade glioma Alteration of the number of copies of double minutes (DMs) with oncogenic EGFR mutations in response to tyrosine kinase inhibitors is a novel adaptive mechanism of glioblastoma. Here we provide evidence that such mutations in DMs, called here amplification-linked extrachromosomal mutations (ALEMs), originate extrachromosomally and could therefore be completely eliminated from the cancer cells. By exome sequencing of seven glioblastoma patients we reveal ALEMs in EGFR, PDGFRA and other genes. These mutations together with DMs are lost by cancer cells in culture. We confirm the extrachromosomal origin of such mutations by showing that wild-type and mutated DMs may coexist in the same tumour. Analysis of 4,198 tumours suggests the presence of ALEMs across different tumour types with the highest prevalence in glioblastomas and low-grade gliomas. The extrachromosomal nature of ALEMs explains the observed drastic changes in the amounts of mutated oncogenes (like EGFR or PDGFRA ) in glioblastoma in response to environmental changes. Human cancers are characterised by the presence of genomic instability [1] , [2] . One form of genomic instability which makes tumours susceptible to acquiring point mutations is often referred to as the mutator phenotype [3] , [4] , [5] . It is expected that the probability of acquisition of gain-of-function mutations in oncogenes is considerably lower than the probability of acquisition of loss-of-function mutations in tumour suppressor genes, because the first occurs in a few critical sites, whereas the latter occurs anywhere in the coding sequence of the gene. Despite that, oncogenes harbour ~80% of the driver mutations [6] . This could be partially explained by the frequent genomic focal amplification (FA) of some oncogenes (that is, RTKs like EGFR, PDGFRA ) [7] , [8] which may increase the probability of acquisition of gain-of-function mutations [9] , [10] , [11] , [12] , [13] , [14] . Several sources of evidence suggest that regions of genomic rearrangements including FAs in cancer may be associated with high mutation loads. In the germline, the DNA mutation loads depend on the number of replication cycles [15] , [16] , and genomic rearrangements frequently coexist with the concomitant mutations [17] . Notably, the break-induced replication repair pathway [18] , [19] was recently suggested to be responsible for the frequent genomic duplications in human cancers [20] . Double minutes (DMs) and homogeneously staining regions (HSR) are the cytogenetic hallmarks of genomic FAs in cancer [21] . DMs are extrachromosomal circular DNA molecules without centromere and are found in the nucleus or cytoplasm enveloped by a nuclear-like membrane (micronuclei) allowing the transcription and DNA replication [22] . The absence of a centromere in DMs results in a random segregation between daughter cells through ‘hitchhiking’ [23] . DMs were found in many tumour types including glioblastomas (GBM) [13] , [24] , low-grade gliomas (LGG), ovary [25] , breast [26] , lung [27] , colon [28] , [29] and neuroblastoma [25] , [30] . The probable mechanism of DM formation involves non-homologous end joining [31] , [32] , [33] which is active in different tumours, especially in those with defective homologous recombination [34] . Therefore the mutation load in DMs is expected to be higher than that in chromosomal DNA, because the repair of DNA damage by non-homologous end joining results in acquisition of point mutations and small indels and the DNA damage repair mechanism is less efficient in the micronuclei compared with the nucleus [29] , [35] . It is also expected that the mutational load in the regions amplified as DMs may be considerably higher than that in the chromosomal non-amplified DNA as this kind of amplification may reach hundreds of copies per cell or more [36] . In this work we describe a novel class of mutations in cancer, amplification-linked extrachromosomal mutations (ALEMs) which occur in DMs. ALEMs are detected in GBMs because they disappear from tumour cells during cell culture. While ALEMs are most prevalent in GBMs and LGG they also exist in other tumour types. Based on these findings, we propose a novel mechanism of acquisition of gain-of-function extrachromosomal mutations mediated by FAs which may underlie the acquisition of resistance to therapies. Amplification-linked mutations We investigated the genetic heterogeneity of GBM by exome sequencing of primary tumour fragments and derived gliomaspheres from seven patients. GBMs were selected for the study, because these tumours are characterised by frequent FAs in their genomes (>50% of the cases) predominantly in the form of DMs [37] . We took advantage of the fact that the cultured GBM spheres in certain conditions can lose DMs [38] , [39] , in order to monitor the fate of point mutations within FAs. 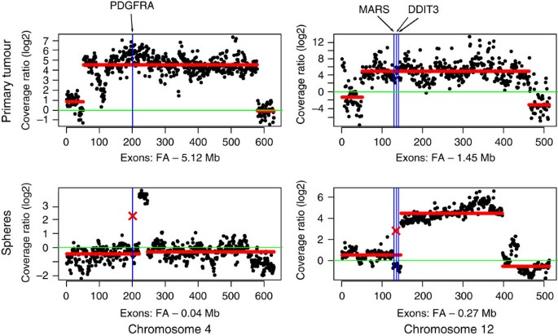Figure 1: Two examples of Focal Amplifications in primary GBM IV-34 in the tumour tissues which are lost in the gliomaspheres. Yaxis- normalised log2 ratios of the sequence coverages between the tumour and the normal samples.Xaxis—equidistantly plotted exons. Green line—diploid state in the tumour. Blue vertical lines depict positions of the mutations. Crosses represent the loss of mutations in gliomaspheres. Red horizontal lines represent hidden Markov models prediction of the regions of amplifications. Focal Amplifications are estimated taking into account the fraction of tumour cells in the tumour samples. We observed eight mutations present within FAs in the primary tumours, and remarkably, all of them were lost in the gliomaspheres after several passages ( Table 1 ). Neither LOH nor chromosomal abnormalities have been detected in the corresponding regions in gliomaspheres. Notably, one individual had four mutations associated with FAs in the primary tumour which were lost in the spheres (GBM IV-34) ( Fig. 1 ). One of these mutations, PDGFRA N659K (COSM22415), was within a 5.1 Mb amplification (chr4:52.86–57.98 Mb), while the other three: MARS p.G888E, DDIT3 p.P11S and DDIT3 p.S31L were within an amplification of 1.5 Mb on chromosome 12 (chr12:57.86–59.31 Mb). The fraction of reads supporting these mutations was close to 100% in the primary tumour sample (86, 97, 99 and 100%, respectively). In addition we performed fluorescence in situ hybridization (FISH) analysis of the interphase nuclei of the GBM IV-34 primary tumour cells and gliomaspheres. The number and localisations of the PDGFRA signals in the primary GBM cells as well as their loss in the cell culture strongly suggests that this FA is present in a form of DMs ( Supplementary Fig. 1a,b ). Table 1 Mutations lost in the spheres and focal amplifications. Full size table Figure 1: Two examples of Focal Amplifications in primary GBM IV-34 in the tumour tissues which are lost in the gliomaspheres. Y axis- normalised log2 ratios of the sequence coverages between the tumour and the normal samples. X axis—equidistantly plotted exons. Green line—diploid state in the tumour. Blue vertical lines depict positions of the mutations. Crosses represent the loss of mutations in gliomaspheres. Red horizontal lines represent hidden Markov models prediction of the regions of amplifications. Focal Amplifications are estimated taking into account the fraction of tumour cells in the tumour samples. Full size image Similar observations were made comparing variants in primary tumours versus spheres from patients GBM IV-19 and GBM IV-39. In both tumours, the EGFR (p.A289V and p.S227Y) mutations and FAs were present in the primary tissues and gliomaspheres at passage 0; however, they were completely lost at later passages ( Table 1 ). The DMs amplifications containing the EGFR locus in the primary tumours and their loss in gliomaspheres in both GBM IV-19 and GBM IV-39 were confirmed by FISH analyses ( Fig. 2 , Supplementary Fig. 1c,d ). 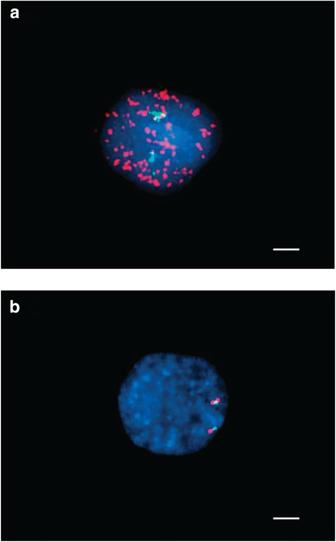Figure 2: FISH analysis for the detection of EGFR amplification in GBM IV-19 cells. (a) FISH in primary tumour cells demonstrates euploid chromosome 7 (green signal) and multiple copies of EGFR scattered all over the nucleus (red signal). (b) Cultured tumour cells shows euploid chromosome 7 in green and not amplified EGFR (red signal). Scale bar=5 μm. Figure 2: FISH analysis for the detection of EGFR amplification in GBM IV-19 cells. ( a ) FISH in primary tumour cells demonstrates euploid chromosome 7 (green signal) and multiple copies of EGFR scattered all over the nucleus (red signal). ( b ) Cultured tumour cells shows euploid chromosome 7 in green and not amplified EGFR (red signal). Scale bar=5 μm. Full size image In addition, we performed metaphase FISH analysis on a GBM cell line (GBM6 kindly provided by Prof. Paul S. Mischel) characterised by strong amplification of the EGFR gene. This cell line is of particular interest as amplified EGFR copies harbour the in-frame deletion of exons 2–7 coding for the extracellular ligand (EGFRvIII) [9] . FISH was performed with probes targeting EGFR and the centromere of chromosome 7. EGFR was present in multiple extrachromosomal copies >100. After culturing with erlotinib in the media, we have repeated the FISH with the same conditions and, in agreement with our previous observations, all extrachromosomal copies have disappeared. Only the chromosomal EGFR was detectable. We have also analysed the data of one patient with GBM reported in the literature [40] , where both the primary tumour tissue and spheres were sequenced. The EGFR p.C326S (COSM1600351) mutation was within the focally amplified region and was identified in 36% of reads of the primary tumour but was lost in the spheres. Mutations of extrachromosomal origin These results raise the question of the origin of the mutations associated with FAs that are present in the primary GBMs and disappear in neurospheres. If mutations associated to FAs are of chromosomal origin and therefore cannot be lost without causing an LOH then their absence in the spheres could be explained by the expansion of a different clone without such mutations ( Fig. 3a lower panel). On the other hand if mutations occur after the formation of DMs and therefore are of extrachromosomal origin, their absence in the spheres could be explained by the loss of DMs from the tumour cells ( Fig. 3a upper panel). In this case, in one cell wild-type DM copies must for some time coexist with DM mutated copies. 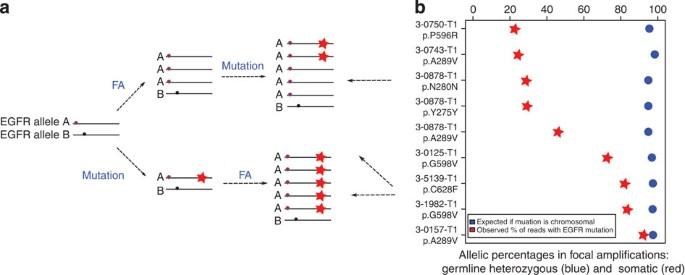Figure 3: Somatic mutations in EGFR occur after focal amplifications in GBM. (a) Models of extrachromosomal mutations (in double minutes) (upper panel) and chromosomal mutation followed by amplification (lower panel). (b) Allelic percentages of heterozygous germline variants and somatic mutations in EGFR focal amplifications. Heterozygous germline variants of allele A and B (blue and black circles); Somatic mutations (red stars). GBM tumours were reanalysed from TCGA consortium. Figure 3: Somatic mutations in EGFR occur after focal amplifications in GBM. ( a ) Models of extrachromosomal mutations (in double minutes) (upper panel) and chromosomal mutation followed by amplification (lower panel). ( b ) Allelic percentages of heterozygous germline variants and somatic mutations in EGFR focal amplifications. Heterozygous germline variants of allele A and B (blue and black circles); Somatic mutations (red stars). GBM tumours were reanalysed from TCGA consortium. Full size image To validate this hypothesis we reanalysed the DNA sequencing data from GBM primary tumours from The Cancer Genome Atlas (TCGA) study [10] with FAs and point mutations in EGFR , focusing on samples where EGFR mutations were present in <90% of reads ( Fig. 3b ). The allelic ratio of the germline heterozygous variants in the tumours was used to estimate the extent of FAs. Cases with suspicion of more than one FA of the EGFR locus were excluded ( Supplementary Fig. 2 ). In the seven remaining TCGA GBM tumours, we detected nine EGFR mutations showing a level of amplification of more than 36 copies per cell. The allelic ratio in these FAs was close to 1 indicating that almost all sequence reads (=>95%) originate from the amplified copies. In addition, four out of nine somatic point mutations in EGFR were present in less than 50% of reads, indicating that a fraction of DM molecules did not contain the mutation ( Fig. 3a upper panel). Therefore, these data confirm the existence of GBM tumours in which the mutated and wild-type DM copies coexist and therefore support the scenario, where the DMs are first formed and the mutation subsequently occurred in one of the DM copies. Thereafter both populations of DM molecules coexist until the DMs carrying the mutation are lost or fixed. We named this new class of mutations as ALEMs. Prevalence of ALEMs in different tumour types In order to investigate the prevalence of co-localisation of FAs and mutations in various tumour types, we investigated 4,198 tumours from 17 tumour types from the TCGA collection, for which both exome sequencing and CNV analyses were performed ( Supplementary Table 1 ). The FAs matching the characteristics of DMs and HSR [31] (more than four copies and length <6 Mb) were included in the study as described in the methods. In total we have identified 1,129 somatic mutations across all tumour types which map within regions of FAs and comprise 0.58% of all studied mutations. We found a positive correlation between mutation rates and extent of FAs across all tumour types ( P =0.002, R =0.75). In each tumour type the mutation rates within FAs were higher than outside, with an average increase of 3.67-fold±2.68. The most important increase of mutation rates within FAs were observed in brain tumours: LGG(9-fold) and GBM (8-fold) ( Fig. 4 ). These tumour types are characterised by frequent FAs in the form of DMs. Since DMs are isolated circular DNA molecules, we hypothesised that a competition between DM copies bearing different somatic mutations may result in positive selection for copies with the strongest oncogenic driver mutation. 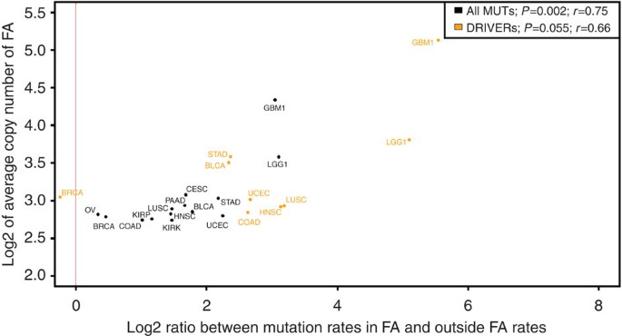Figure 4: Correlation of increase of mutation rates in FAs with the FA copy number. Statistical significance was assessed with analysis of variance.Xaxis—log2 of the ratio between mutations rates inside FAs and outside.Yaxis—log2 of the average copy number in FAs. Each data point represents the tumour type. Black—all mutations (N=14). Orange—mutations in oncogenes (N=9). Red line represents equal mutations rates inside and outside of FAs. Figure 4: Correlation of increase of mutation rates in FAs with the FA copy number. Statistical significance was assessed with analysis of variance. X axis—log2 of the ratio between mutations rates inside FAs and outside. Y axis—log2 of the average copy number in FAs. Each data point represents the tumour type. Black—all mutations ( N =14). Orange—mutations in oncogenes ( N =9). Red line represents equal mutations rates inside and outside of FAs. Full size image To test this hypothesis, we generated a data set of mutations enriched in oncogenic driver mutations in 54 documented oncogenes [6] . Remarkably 27% of all ‘oncogenic’ driver mutations were located within FAs. The probability of fixation of ‘oncogenic’ driver mutations in FAs as compared with the total number of mutations increased in almost all tumour types with the most pronounced effect in LGG (4-fold ) and GBM (6-fold). A similar result was obtained in a different data set enriched in putative driver mutations, where only mutations with at least three occurrences in the COSMIC v67 database ( Supplementary Fig. 3 ) were included. Interestingly, when a similar analysis was performed with only passenger mutations, many of these were also localised with FAs in all tumour types, however with a smaller enrichment compared with what was observed with putative driver mutations ( Supplementary Fig. 3 ). Next we investigated which genes exhibit non-random co-localisation of mutations with FAs. When all tumours were analysed, 212 genes revealed a significant enrichment of mutations in focally amplified regions ( P <0.05). This list of genes included RTK such as EGFR, PDGFRA, ERBB2 and KIT ; other receptors associated to cancer such as NOTCH3 , EPHA6 and other oncogenes including CCNE1, BCL11A, WHSC1L1 and CDK8 ( Supplementary Data 1 ). We reasoned that genes mapping near known drivers found in FAs, may also display increased mutation rate. We observed this effect in MED1 which is located 0.25 Mb from ERBB2 ; and in SHANK2 and PPFIA1 genes near CCND1 (0.84 and 0.65 Mb, respectively) which is known to be amplified in a form of DMs [27] , [39] , [41] , [42] , [43] , [44] , [45] . These closely located genes on the chromosome are likely to be co-amplified in the same FA ( Fig. 5 ). 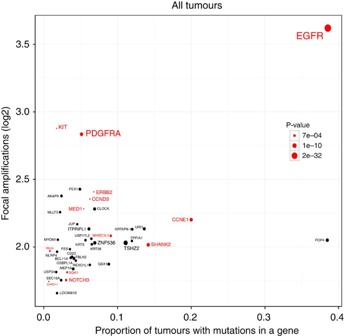Figure 5: Co-localisations of mutations and amplifications on gene-by-gene basis across 17 tumour types andN=4,198 tumour samples. Xaxis—proportion of mutations in Focal Amplifications,Yaxis—log2 of the average copy number in FAs. The area in circle is inversely proportional to the log2 of the log2 of theP-value (Fisher test). All oncogenes are selected in red. All oncogenes are presented if they have at least one mutation in FAs and aP-value less than 0.15, the other genes are presented if they have at least two mutations in FAs andP-value less than 0.01. Figure 5: Co-localisations of mutations and amplifications on gene-by-gene basis across 17 tumour types and N =4,198 tumour samples. X axis—proportion of mutations in Focal Amplifications, Y axis—log2 of the average copy number in FAs. The area in circle is inversely proportional to the log2 of the log2 of the P -value (Fisher test). All oncogenes are selected in red. All oncogenes are presented if they have at least one mutation in FAs and a P -value less than 0.15, the other genes are presented if they have at least two mutations in FAs and P -value less than 0.01. Full size image To reveal tumour-specific oncogenes that exhibit the pattern of co-localisation of mutations within FAs, we repeated the gene-by-gene analyses independently per each tumour type. The strongest enrichment of mutations in FAs was observed in EGFR in GBM, low-grade glioma, head and neck squamous-cell carcinoma, lung and uterine cancer. PDGFRA mutations were enriched in FAs in GBM, low-grade glioma and lung cancer; and KIT mutations in lung cancer. Similar co-localisations were observed for NOTCH3 mutations in ovarian and breast cancers; CCNE1 mutations in uterine cancer; BCL11A mutations in lung cancer and WHSC1L1 mutations in head and neck squamous-cell carcinoma and lung cancer ( Supplementary Fig. 4 ). The fraction of putative driver mutations that occurred in FAs was increased for all tested oncogenes. The most remarkable effect was observed in EGFR where the percentage of mutations in FA in all tumours increased from 39% (all mutations) to 65% (putative driver mutations) followed by PDGFRA (from 17 to 50% in LGG) and ERBB2 (from 7 to 11% in all tumours). These results taken together suggest a positive selection for DM clones carrying oncogenic driver mutations. In this work we demonstrate the existence of a non-random association of FAs and likely driver mutations in tumours. In addition, we propose a mechanism for acquisition of gain-of-function driver mutations in oncogenes mediated by the higher mutation load observed in DMs. In several independent cases from this study and from Yost et al. [40] , both amplifications and mutations present in the primary GBM tumours were lost during cell culturing suggesting their extrachromosomal origin. DM origin of such mutations was confirmed by revealing the GBM tumours where wild type and mutated DM copies coexist ( Fig. 3a upper panel). We hypothesise that this phenomenon is taking place in several steps. The process begins with the generation of the DM molecules, which may happen in an almost random fashion across the genome. When the increased number of copies of a gene provides a proliferative advantage to the tumour cell, this event has a probability of being expanded in the tumour. The amplified DNA region is prone to acquisition of an increased number of variants because of a higher number of DNA copies (similar mutation rates with corresponding locus of genomic DNA) or a higher rates of acquisition of variants (higher mutation rates than in the corresponding locus of genomic DNA) or a combination of both. Subsequently, DMs with the oncogenic variants may be subjected to selection based on the random distribution of DMs among daughter cells. After cell division the cell with the highest number of DMs harbouring the driver mutation will have a proliferative advantage. The end point of this process is the presence of a high number of DMs per cell, where almost all copies have the driver ALEMs ( Fig. 6 ). 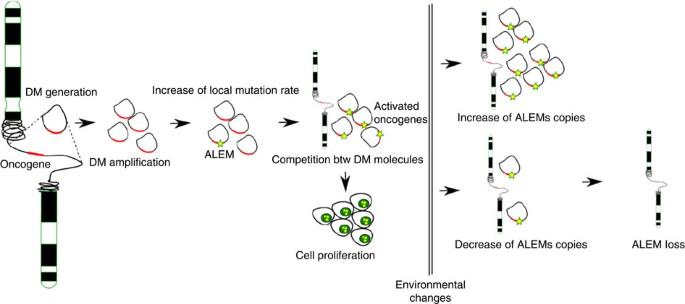Figure 6: Model of generation and function of ALEMs. After random generation of the DM molecules, the amplified DNA region is prone to acquisition of an ALEM due to a higher number of DNA copies. The cell with the highest number of DMs harbouring the ALEM will have a proliferative advantage. In response to environmental stress the cells may accordingly change the amount of DMs (see text for details). Figure 6: Model of generation and function of ALEMs. After random generation of the DM molecules, the amplified DNA region is prone to acquisition of an ALEM due to a higher number of DNA copies. The cell with the highest number of DMs harbouring the ALEM will have a proliferative advantage. In response to environmental stress the cells may accordingly change the amount of DMs (see text for details). Full size image An important consequence of this model is that, in the case of changes of environmental conditions, the number of DMs could be modulated and even reduced to zero resulting in the complete loss of ALEMs. The same mechanism would not be possible if these amplifications were in a form of HSR. Indeed the selection and competition between copies of amplified DNA with different genetic background is only possible between spatially isolated molecules, such as in the case of DMs. Moreover strong gain-of-function mutations in HSR amplifications would be detectable only if they have occurred at the early steps of amplification and were found in a high proportion of copies. Another consequence of this model observed in this study is the enrichment of passenger mutations in FAs which can be explained by the ‘hitchhiking’ effect. By studying a large number of tumours from publicly available data (TCGA consortium), we have detected co-localisation of mutations with amplifications in tumours known to harbour DMs such as GBM, LGG and LUSC [13] , [24] , [27] . Interestingly, genes highly affected by ALEMs were members of RTK family, such as EGFR , PDGFRA and ERBB2 . We also noted that driver ALEMs were 26-fold more frequent in GBM and 13-fold in LGG than the passenger ALEMs. These two facts confirm the expected positive selection for the driver mutations in DMs. Remarkably, our model explains the observations made by Nathanson et al. [9] , where the extrachromosomal EGFRvIII mutation disappeared in response to tyrosine kinase inhibitors. ALEMs may make tumour cells fast-adaptable to the environmental changes including those induced by anticancer treatments. For example, we speculate that this mechanism may be utilised to acquire resistance to vemurafenib treatment in the BRAF V600E positive tumours [46] . According to our model amplification of EGFR which is not a strong oncogenic event per se [47] , [48] , [49] , [50] may increase the mutation load and enhance the probability of acquisition of the driver mutations in EGFR . In conclusion, we provide evidence to support a novel type of cancer variants, the ALEMs. They result from a mutagenic process which is based on the increased mutational load of DMs that include proliferation-promoting genes such as tyrosine-kinases receptors leading to an increased adaptive potential of the tumour cells. Processing of tumours and gliomasphere cultures In patient samples, tumour resections were obtained after surgery at the University Hospital of Geneva. After approval of the ethics committee of the Geneva University Hospitals informed written consent was obtained for all subjects. Primary tumour samples were cut in pieces and fresh frozen until analysis. Human biopsies were chopped mechanistically and digested with papain and DNase to generate a cell suspension. Gliomaspheres were thereof generated as previously described [51] . Briefly, media (DMEM-F12, B27 2%) and growth factors (EGF and bFGF at 10 ng ml −1 ) were renewed once every 5 days. Peripheral blood was obtained at the time of surgery. Peripheral blood mononuclear cells were isolated over a Ficoll gradient and frozen in liquid nitrogen in 10% DMSO until analysis. DNA extraction and exome sequencing The overall methodology was as previously described [52] , [53] , [54] . Briefly, DNA was extracted from the two distant fragments of frozen tissues, neurosphere cultures (spheres) and peripheral blood lymphocytes using the QIAamp DNA Mini Kit (Qiagen) for seven patients with GBM. When little material was available (<0.5 μg), Whole genome amplification was performed using REPLI-g Mini Kit (Qiagen). Exome capture was conducted using the SureSelect Human Exon v3 50 Mb (Agilent Technologies) reagents and sequencing was performed on Illumina HiSeq2000 instrument (Illumina) with paired-end 105 nt reads. Burrows–Wheeler Aligner (BWA) software [55] was used to align the sequence reads to the human reference genome (NCBI build GRCh37/hg19). SAMtools [56] was used to remove polymerase chain reaction (PCR) duplicates and to call single-nucleotide variants (SNV). Detection of small insertions and deletions (smINDEL) was conducted with Pindel 0.2.2 software [57] . The average sequencing coverage was 155 × per DNA sample ( Supplementary Table 2 ). The search for somatic mutations was restricted to the regions covered at least 20-fold in both the normal and tumour samples. Calling of SNVs The initial list of SNVs was filtered against the common (>1%) germline polymorphisms present in the dbSNP137 and 1,000 genomes databases. SNVs present in the normal tissue sample from the same patient at a frequency of >1% were also filtered out. In contrast to the SNVs, smINDELs were called with lower accuracy and, therefore, we report only those smINDELs that were validated by Sanger sequencing. For both SNVs and smINDELs, we focused on the mutations that map to the protein coding sequences and to splice sites, as the untranslated exonic regions were less well covered by the commercially available exome capture reagents used in this study ( Supplementary Data 2 ). Calling of LOHs and focal amplifications Two sources of information from exome sequencing were used to estimate the somatic copy number alterations: (i) the fractions of reads with the heterozygous germline variants; and (ii) the ratios of the coverage of the tumour sample and the corresponding normal DNA. An in-house hidden Markov models based algorithm was used to predict the regions of FAs taking into account both sources of data. FAs were confirmed with quantitative PCR ( Supplementary Fig. 5 ). Primers for quantitative PCR are reported in the Supplementary Table 3 . FISH analysis Genes amplifications were investigated by FISH analysis using the LSI EGFR Spectrum Orange/CEP7 Spectrum Green probe (Vysis, Abbott Laboratories, IL, USA) and the BAC probe RP11-231c18 directed against PDGFRA (chr4:55,127,335-55,259,498; hg19, spectrum green) and the control probe dj963K6 (4qter, spectrum red). The FISH signals for each locus-specific FISH probe were assessed under an Zeiss Axioscop microscope (Zeiss) equipped with specific filters (DAPI/Green/Red). DAPI II (4,6-diamino-2-phenyindole-2-hydrochloride) was used for chromatin counterstaining. TCGA data analysis The tumours for which exome-sequencing and CNV data were publicly available in TCGA [10] were analysed in this study ( Supplementary Table 1 ). When several kinds of SNV analyses were available for the same tumours, we selected those which covered the largest number of samples. We selected amplifications of more than 4-fold and length less than 6 Mb [31] . The Fisher exact test was applied for statistical assessment of non-random co-localisation of FAs and point mutations. Accession codes: Sequence data for exome-sequencing of primary tumour fragments, matched blood samples and derived gliomaspheres have been deposited in GenBank/EMBL/DDBJ under the accession code PRJNA263837 . How to cite this article : Nikolaev, S. et al. Extrachromosomal driver mutations in glioblastoma and low grade glioma. Nat. Commun. 5:5690 doi: 10.1038/ncomms6690 (2014).